Facile scission of isonitrile carbon–nitrogen triple bond using a diborane(4) reagent Transition metal reagents and catalysts are generally effective to cleave all three bonds (one σ and two π ) in a triple bond despite its high bonding energy. Recently, chemistry of single-bond cleavage by using main-group element compounds is rapidly being developed in the absence of transition metals. However, the cleavage of a triple bond using non-transition-metal compounds is less explored. Here we report that an unsymmetrical diborane(4) compound could react with carbon monoxide and tert -butyl isonitrile at room temperature. In the latter case, the carbon–nitrogen triple bond was completely cleaved in the absence of transition metal as confirmed by X-ray crystallographic analysis, 13 C NMR spectroscopy with 13 C labelling and DFT calculations. The DFT calculations also revealed the detailed reaction mechanism and indicated that the key for the carbon–nitrogen triple-bond cleavage could be attributed to the presence of nucleophilic nitrogen atom in one of the intermediates. A triple bond having three shared electron pairs between two atoms is known as one of the strongest chemical bonds. In spite of the large bonding energy, complete cleavage of the three (one σ and two π ) bonds in a C≡C triple bond of an alkyne molecule or in a C≡N triple bond of a nitrile molecule under oxidative or acidic condition is common in general organic chemistry. In addition to the well-established chemistry of alkyne metathesis [1] , some stoichiometric [2] , [3] , [4] and catalytic [5] , [6] , [7] , [8] , [9] , [10] , [11] reactions for complete cleavage of a C≡C triple bond are also known with transition metal (TM) reagents and catalysts. However, only two examples about the cleavage of a C≡C triple bond without TMs have been reported using tandem- and multi-step reactions under harsh condition [12] , [13] . Moreover, cleavage of the C≡O triple bond in carbon monoxide (CO) is widely known as the Fischer–Tropsch process in the presence of a TM catalyst [14] . Recent development of TM catalysts enabled us to cleave the N≡N triple bond in dinitrogen for the formation of ammonia [15] , [16] , [17] . Several catalytic [18] and stoichiometric [19] , [20] cleavage reactions of a C≡N triple bond were also reported with use of TM catalyst and reagent [21] , [22] , [23] . Although some p-block element compounds could also react with CO [24] , [25] , [26] , [27] , [28] , [29] , [30] , [31] , [32] , [33] , [34] , [35] , [36] , [37] , [38] or isonitriles [28] , [39] , [40] , the strongest σ -bond among the three bonds in a triple bond remained intact in all cases. On the other hand, chemistry containing Lewis-base adduct of sp 2 – sp 3 diborane(4) compounds has been quickly developed recently. After the isolation of the first example of base adduct of bis(catecholato)diborane(4) [41] , [42] , [43] , [44] , [45] , a series of the sp 2 – sp 3 diborane(4) compounds were applied as a boron source for copper-catalysed β-borylation of α,β-unsaturated carbonyl compounds in the absence of additional base [46] , [47] , [48] , as a hydrogen donor for radical reduction [49] and as reactive compounds to undergo rearrangement reactions [50] , [51] , [52] , [53] . Some Lewis-base-catalysed β-borylation reactions of α,β-unsaturated carbonyl compounds were also considered to involve such sp 2 – sp 3 diborane(4) intermediates [54] , [55] , [56] , [57] , [58] , [59] , [60] , [61] . Herein, we report a complete cleavage reaction of C≡N triple bond in isonitrile by using unsymmetrical diborane(4) compound, involving sp 2 – sp 3 diborane(4) intermediates supported by density functional theory (DFT) calculations. Synthesis and reactivity of diborane(4) with CO and t BuNC Synthesis of the unsymmetrical diborane(4) 2 , its reactions and characterization of the resulting products are summarized in Fig. 1 (see also, Supplementary Figs 1–15 , Supplementary Tables 1 and 2 , and Supplementary Methods ). Reaction of 1 with mesitylmagnesium bromide gave 2 in 49% yield. The 1 H NMR spectrum of 2 showed C 2v symmetrical pattern of signals. Two broad 11 B NMR signals were observed at δ B 34 and 89 p.p.m., indicating the selective conversion of one (pinacolato)boryl group to a dimesitylboryl group. Broadening of a 13 C NMR signal at δ C 144.2 p.p.m. also confirmed the connection between the mesityl groups and a quadrupolar boron nucleus. X-ray crystallographic analysis of 2 revealed twisted orientation described by the dihedral angle of O1–B1–B2–C16 in contrast to the case of 1 ( Supplementary Fig. 16 ) [62] . DFT calculation showed that the vacant p -orbital of the boron atom in the Bpin moiety slightly contribute to the LUMO of 2 ( Supplementary Figs 17–18 ), which mainly consisted of the vacant p-orbital of the boron atom in the BMes 2 moiety, in spite of the twisted structure. 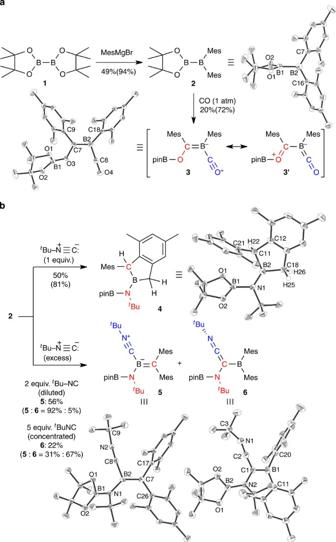Figure 1: Synthesis and reactions of unsymmetrical diborane(4)2. (a) Synthesis and reaction of2with CO to form3and their crystal structures. (b) Reaction of2towardstert-butylisonitrile to form4–6and crystal structures of the products (isolated and1H NMR yield in parentheses, Mes=2,4,6-(CH3)3C6H2, pinB=[(CH3)2CO]2B): Selected bond lengths (Å), bond angles (°) and dihedral angles (°);2: B1–B2=1.722(4);3: B1–O1=1.366(3), B1–O2=1.356(3), B1–O3=1.374(3), O3–C7=1.406(3), C7–B2=1.459(4), B2–C8=1.492(4), C8–O4=1.144(3);4: B1–N1=1.455(3), N1–B2=1.415(3), B2–C11=1.626(4), B2–C18=1.591(4);5: B1–N1=1.413(3), N1–B2=1.495(3), B2–C7=1.456(3), B2–C8=1.569(3), C8–N2=1.152(3), B2–C8–N2=173.6(2);6: B1–C1=1.516(7), C1–C2=1.353(6), C2–N1=1.217(5), C1–N2=1.450(5), B2–N2=1.419(6), B1–C1–C2=114.8(4), C1–C2–N1=174.5(5), C2–N1–C3=131.7(4). Figure 1: Synthesis and reactions of unsymmetrical diborane(4) 2 . ( a ) Synthesis and reaction of 2 with CO to form 3 and their crystal structures. ( b ) Reaction of 2 towards tert -butylisonitrile to form 4 – 6 and crystal structures of the products (isolated and 1 H NMR yield in parentheses, Mes=2,4,6-(CH 3 ) 3 C 6 H 2 , pinB=[(CH 3 ) 2 CO] 2 B): Selected bond lengths (Å), bond angles (°) and dihedral angles (°); 2 : B1–B2=1.722(4); 3 : B1–O1=1.366(3), B1–O2=1.356(3), B1–O3=1.374(3), O3–C7=1.406(3), C7–B2=1.459(4), B2–C8=1.492(4), C8–O4=1.144(3); 4 : B1–N1=1.455(3), N1–B2=1.415(3), B2–C11=1.626(4), B2–C18=1.591(4); 5 : B1–N1=1.413(3), N1–B2=1.495(3), B2–C7=1.456(3), B2–C8=1.569(3), C8–N2=1.152(3), B2–C8–N2=173.6(2); 6 : B1–C1=1.516(7), C1–C2=1.353(6), C2–N1=1.217(5), C1–N2=1.450(5), B2–N2=1.419(6), B1–C1–C2=114.8(4), C1–C2–N1=174.5(5), C2–N1–C3=131.7(4). Full size image The unsymmetrical diborane(4) 2 reacted with CO or t BuNC to give a variety of products ( Fig. 1 ). A benzene solution of 2 was exposed to CO at room temperature for 30 min to give pale yellow solids of 3 in 20% isolated yield. X-ray crystallography for 3 showed incorporation of two CO molecules (it should be noted the complete assignment of atomic order in 3 , 5 and 6 would be difficult due to small difference in electron density of the second period elements; see below and Fig. 2 ). The O3–C7 [1.406(3) Å], C7–B2 [1.459(4) Å] and B2–C8 [1.492(4) Å] bonds are shorter than the conventional single bonds, and C8–O4 [1.144(3) Å] is slightly longer than the C≡O bond of free CO molecule (1.1283 Å) [63] . These data proposed resonance structures of 3 and 3' with a characteristic conjugated O–C–B–C–O linkage giving a pale yellow colour ( Supplementary Fig. 19 for ultraviolet–visible spectrum and Supplementary Tables 3 and 4 for time-dependent DFT calculation). Thus, compound 3 could be described as CO-coordinated alkoxyboraalkene. Reaction of 2 with one equivalent of t BuNC gave a colourless cyclized product 4 in 50% yield through scission of the isonitrile C≡N triple bond and of a C(sp 3 )–H bond in one of the mesityl substituents, as the molecular structure of 4 was confirmed by X-ray crystallographic analysis. The assignment of the B2 atom in the 2-boraindane skeleton could also be supported by the relatively long B2–C11 [1.626(4) Å] and B2–C18 [1.591(4) Å] bonds. In contrast, the reaction of 2 with an excess amount of t BuNC gave a mixture of t BuNC-coordinated boraalkene 5 and borylethenylideneamine 6 . The reaction with two equivalents of t BuNC in a diluted solution gave 5 as the major product, while the reaction with a large excess amount of t BuNC in a concentrated solution afforded 6 as the major product. X-ray crystallographic analysis of 5 and 6 revealed that these two compounds have similar arrangement of all atoms, except the order of the two atoms in the central B=C or C–B bond and the terminal C–N– t Bu angle ( 5 , B2–C8–N2=173.6(2)°; 6 , C2–N1–C3=131.7(4)°). To form 5 , the C≡N triple bond in t BuNC, one B–B bond and two B–Mes bonds were cleaved from 2 , while the two mesityl groups are still attached to the boron atom in 6 . In the molecular structure of 5 , the boron centre has B=C double-bond character (B2–C7=1.456(3) Å) and the second equivalent of t BuNC coordinates to the boron atom in the B=C moiety. In the case of 6 , the t BuNC moiety has consecutive N=C and C=C double bonds (N1=C2=1.217(5) Å, C2=C1=1.353(6) Å) with a slightly short C–B single bond (C1–B1=1.516(7) Å). All the obtained crystal structures could be reproduced by DFT calculation to support the assignment of atomic order (see below). 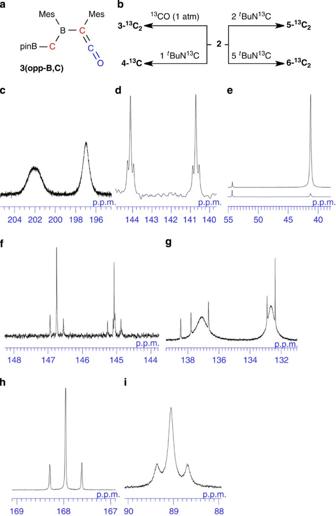Figure 2: Assignment of atomic order in3–6by13C NMR experiments with13C labelling. (a) Potential regioisomer3(opp-B,C)derived from exchange of the positions of boron and carbon atoms in3. (b) Reactions of2with13C-labelled13CO andtBuN13C to form the corresponding13C-labelled3-13C2,4-13C,5-13C2and6-13C2. (c) Newly appeared13C NMR signals of3-13C2on13C labelling. (d) The 4° aromatic signals of4-13Cwith satellite on13C labelling (e) enhancement of13C NMR signal (top:4-13C, bottom:4). (f) The 4° aromatic signals of5-13C2with satellite on13C labelling (g) newly appeared13C NMR signals of5-13C2on13C labelling (h). (i) Strengthened13C NMR signals of6-13C2with satellite on13C labelling. Figure 2: Assignment of atomic order in 3 – 6 by 13 C NMR experiments with 13 C labelling. ( a ) Potential regioisomer 3(opp-B,C) derived from exchange of the positions of boron and carbon atoms in 3 . ( b ) Reactions of 2 with 13 C-labelled 13 CO and t BuN 13 C to form the corresponding 13 C-labelled 3- 13 C 2 , 4- 13 C , 5- 13 C 2 and 6- 13 C 2 . ( c ) Newly appeared 13 C NMR signals of 3- 13 C 2 on 13 C labelling. ( d ) The 4° aromatic signals of 4- 13 C with satellite on 13 C labelling ( e ) enhancement of 13 C NMR signal (top: 4- 13 C , bottom: 4 ). ( f ) The 4° aromatic signals of 5- 13 C 2 with satellite on 13 C labelling ( g ) newly appeared 13 C NMR signals of 5- 13 C 2 on 13 C labelling ( h ). ( i ) Strengthened 13 C NMR signals of 6- 13 C 2 with satellite on 13 C labelling. Full size image The NMR spectroscopic characterization of the products The nuclear magnetic resonance (NMR) spectra of 3 – 5 were consistent with the crystallographically determined structures. The 1 H NMR spectrum of 3 in C 6 D 6 showed two distinct Mes groups and one pinacol moiety. Two boron nuclei resonated at δ B –5 and 18 p.p.m., where the former signal could be assigned as the CO-coordinated boron atom due to the negatively charged boron atom in both the resonance structures 3 and 3′ . The calculated 11 B NMR chemical shift ( δ B –4.1, 20 p.p.m.) of 3 by the Gauge-independent atomic orbital (GIAO) method at B3LYP/6-311++G(2d,p)//B3LYP/6-31+G(d,p) level was also in good agreement with the experimental data ( Supplementary Table 5 ). Although the two Mes groups and the pinacol moiety could be assigned in the 13 C NMR spectrum of 3 , no signal corresponding to a B=C unit and a coordinating CO molecule was observed. The 1 H NMR spectrum of 4 showed one benzylic methine proton ( δ H 4.22) and two vicinally coupled methylene protons ( δ H 2.87 and 2.93, 2 J HH =21 Hz), supporting the scission of a C( sp 3 )–H bond in one of the two mesityl groups to give a chiral centre on C11. Reflecting the asymmetry below and above the 2-boraindane plane in 4 , all the remaining five methyl groups on the mesityl substituents were separately observed and the four methyl groups on the pinacolato moiety resonated two singlet signals. Both the boron nuclei in 4 resonated at a typical region for an sp 2 boron atom ( δ B 27, 55 p.p.m.). The lower-field shifted signal could be assigned as the dicarbyl-substituted boron atom as supported by our GIAO calculations. Two relatively broadened 13 C NMR signals at δ C 30.3 and 41.2 p.p.m., compared with other signals of 4 , supported their connection to quadrupolar boron nucleus. The 1 H NMR spectra of 5 and 6 similarly showed six methyl signals for the Mes groups, two methyl signals for the pinacol moiety, two t Bu signals and four aromatic CH signals, because they are regioisomers with the same combination of the substituents and are close in symmetry of molecule. In the 13 C NMR spectrum of 5 , the number of observed signals was two short of the number of 13 C nuclei expected from the symmetry of the 1 H NMR spectrum. Similarly, one carbon signal was missing in the 13 C NMR spectrum of 6 . The missing of the 13 C signals was probably due to broadening of quaternary carbon bonded to quadrupolar boron nucleus. The 11 B NMR signals of 5 ( δ B 13, 21 p.p.m.) and 6 ( δ B 21, 63 p.p.m.) could also be assigned by our GIAO calculations. The 13 C-labelling study to determine the atomic order In addition to the conventional NMR spectra of 3 – 5 , 13 C-labelling experiment could confirm the structures of 3 – 6 including connectivity between boron and carbon atoms ( Fig. 2 ). Complete structural characterization of 3 , 5 and 6 was difficult due to the following reasons: (1) in general, X-ray crystallographic analysis has difficulty to distinguish two adjacent atoms in the same row of the periodic table. This means that positions of carbon and boron atoms in 3 versus 3(opp-B,C) ( Fig. 2a ) and 5 versus 6 could not be unambiguously determined by crystallography. (2) Both 10 B and 11 B nuclei are quadrupolar to induce significant broadening of the signal for boron-bonded nuclei, leading in difficulty for observation of quaternary carbon bonded to boron nucleus. In this context, we performed 13 C-labelling experiments for 3 – 6 to observe the 13 C– 13 C coupling and broadened 13 C NMR signals bonded to boron atom. The unsymmetrical diborane 2 reacted with 13 C-labelled 13 CO (99% 13 C) or t BuN 13 C (20% 13 C) gave 13 C-labelled 3- 13 C 2 , 4- 13 C , 5- 13 C 2 and 6- 13 C 2 ( Fig. 2b ). On 13 C-labelling of 3 , two broad signals at δ C 197.1 and 201.8 p.p.m. appeared without apparent coupling in the 13 C NMR spectrum of 3- 13 C 2 ( Fig. 2c ), indicating that these two carbon atoms connected to a quadrupolar boron atom with the C–B=C skeleton in 3 (not C–C=B in 3(opp-B,C) ). As described above, two broadened signals δ C 30.3 and 41.2 p.p.m. may be assigned to the boron nucleus in 4 . The lower-field shifted signal at δ C 41.2 p.p.m. was strengthened on 13 C labelling to form 4- 13 C ( Fig. 2e ), indicating this benzylic methine carbon came from t BuN 13 C. Concomitantly, two signals of aromatic quaternary carbons at δ C 140.7 and 144.1 p.p.m. were accompanied with satellite signal with 1 J CC of 40 Hz ( Fig. 2d ), similar to that (43 Hz) for the C( sp 2 )–C( sp 3 ) linkage in strychnine [64] , indicating that the two ipso carbons of the two Mes groups bonded to the sp 3 methine 13 C are from t BuN 13 C. In the case of 5- 13 C 2 , two broad signals appeared at δ C 132.7 and 137.1 p.p.m. on labelling ( Fig. 2g ), supporting the C–B=C skeleton of 5 . Two split 4° aromatic signals with 1 J CC of 24 Hz in 5- 13 C 2 also showed that the two Mes groups bonds to a carbon atom ( Fig. 2f ). The 13 C NMR spectrum of 6- 13 C 2 showed two strengthened signals at δ C 89.1 and 168.0 p.p.m. ( Fig. 2h,i ) with a satellite ( 1 J CC =86 Hz), supporting the C( sp 2 )–C( sp ) coupling (107 Hz in diphenylketene- 13 C 2 ) [65] . One can confirm that the carbon atom with the δ C 89.1 p.p.m. signal is bonded to a quadrupolar boron atom in the structure of 6 , according to the broadening observed. Proposed mechanism based on DFT calculation The whole mechanisms for the formation of 3 – 6 from 2 were estimated by DFT calculations [66] , [67] , [68] , [69] with full geometry optimization of all the available transition states (TSs) at the B3LYP/6-31G(d,p) level and single-point energy calculation at M06-2X/6-311+G(d,p) with solvent effect of benzene using conductor-like polarizable continuum model ( Fig. 3 : mechanism with curly arrows, Fig. 4 : energy profiles with relative Gibbs free energies and Supplementary Table 6 for coordinates of all the structures). An initial coordination of CO or t BuNC to 2 gave the sp 2 – sp 3 diborane(4) 7-O and 7-N , which would undergo two types of bond cleavage reactions ( Fig. 3a ): (1) B–Mes bond cleavage to give acyldiborane(4) 8-O or imidoyldiborane(4) 8-N , (2) B–Bpin bond cleavage to give diborylketone 9-O or diborylimine 9-N . In the reaction of 2 with CO, energy levels of TS8-O and TS9-O are comparable to each other and both TSs are higher than the TS7-O ( Fig. 4a ). The slightly lower TS8-O could be explained by the higher nucleophilicity of a Mes substituent than a Bpin substituent due to the electronegativity difference between carbon and boron atoms, as supported by natural bond orbital analysis ( Supplementary Fig. 20 ). The subsequent reactions from 8-O and 9-O afforded the same product 3 ( Fig. 3b ). The former pathway through 8-O included a coordination of a second CO molecule to give 10-O and subsequent migration of the Bpin moiety by a nucleophilic attack of the acyl oxygen atom in 10-O with B–B bond cleavage to give 3 . The large energy gain in this step may be attributed to the formation of B–O bond. The latter pathway through 9-O was initiated by a Bpin migration to form the borataalkene 11-O . TS11-O was the global TS, which lies 6.1 kcal mol −1 higher than TS8-O . Subsequently, one of the two Mes groups in 11-O migrated to the carbon atom to afford the boraalkene 12-O . Coordination of a second CO molecule to 12-O could form the same product 3 . This step could be considered as a coordination of CO to electron-deficient boraalkene for a large energy gain. Formation of a possible C–O cleaved product 13-O would be suppressed due to the higher TS13-O ( Fig. 4a ). 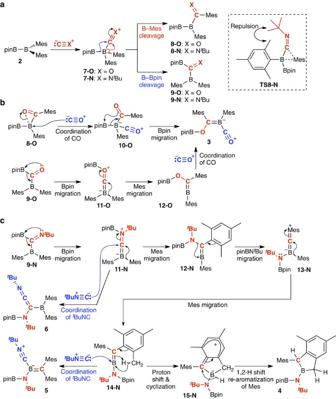Figure 3: Possible reaction mechanism for the formation of3–6from2estimated by DFT calculations. (a) Two types of possible products8and9formed by B–Mes or B–Bpin cleavage after the coordination of CO ortBuNC. (b) Two energetically comparable pathways to3from8-Oand9-O. (c) Three pathways to4-6from9-N. Figure 3: Possible reaction mechanism for the formation of 3 – 6 from 2 estimated by DFT calculations. ( a ) Two types of possible products 8 and 9 formed by B–Mes or B–Bpin cleavage after the coordination of CO or t BuNC. ( b ) Two energetically comparable pathways to 3 from 8-O and 9-O . ( c ) Three pathways to 4 - 6 from 9-N . 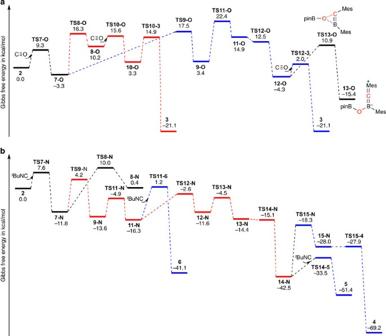Figure 4: Energy profiles of possible mechanism. Energy profiles of possible mechanism for the formation of3–6from2with relative Gibbs free energies in kcal mol−1(estimated by optimization at the B3LYP/6-31G(d,p) level and subsequent single-point energy calculation at M06-2X/6-311+G(d,p) level with consideration of entropy contribution and solvent effect of benzene (conductor-like polarizable continuum model (CPCM)), all the compound numbers are in conjunction withFig. 3). (a) Two possible pathways for the formation of3by reaction of2with CO (red: pathway through8-O, blue: pathway through9-O) (b) pathway for the formation of4-6by reaction of2withtBuNC (red: main pathway to4-6, blue: branching to each of the compounds4-6). (Remark: before the solvation correction,TS12-Ois slightly higher than11-OandTS14-Nis slightly higher than13-Nin energy.) Full size image Figure 4: Energy profiles of possible mechanism. Energy profiles of possible mechanism for the formation of 3 – 6 from 2 with relative Gibbs free energies in kcal mol −1 (estimated by optimization at the B3LYP/6-31G(d,p) level and subsequent single-point energy calculation at M06-2X/6-311+G(d,p) level with consideration of entropy contribution and solvent effect of benzene (conductor-like polarizable continuum model (CPCM)), all the compound numbers are in conjunction with Fig. 3 ). ( a ) Two possible pathways for the formation of 3 by reaction of 2 with CO (red: pathway through 8-O , blue: pathway through 9-O ) ( b ) pathway for the formation of 4-6 by reaction of 2 with t BuNC (red: main pathway to 4-6 , blue: branching to each of the compounds 4-6 ). (Remark: before the solvation correction, TS12-O is slightly higher than 11-O and TS14-N is slightly higher than 13-N in energy.) Full size image In the reaction of 2 with t BuNC, TS8-N was 5.8 kcal mol −1 higher than TS9-N , indicating that the pathway through 9-N would be favourable ( Fig. 4a ). The high energy level of TS8-N may be explained by a steric repulsion between the spectator Mes group and the t Bu group ( Fig. 3a and Supplementary Table 7 ). The intermediate 9-N would undergo Bpin migration to give 11-N followed by a Mes group migration to form the boraalkene 12-N ( Fig. 3c ). Coordination of t BuNC to the central carbon atom in 11-N could lead to formation of 6 , but the TS to 6 was calculated to be slightly higher (by 3.8 kcal mol −1 ) than the TS to 12-N . Requirement of higher concentration to prepare 6 was consistent with this result. Again, the simple coordination of t BuNC to boraalkene would give a large energy gain. As a nitrogen atom in 12-N may have higher nucleophilicity than the oxygen atom in 12-O , a migration of the amino substituent (−N t BuBpin) to the Mes-bonded boron atom would take place with an assistance of electron donation from the carbon-bonded Mes group to form the amino-substituted borataalkene 13-N . This step (from 12-N to 13-N ) involves a cleavage of the C–N bond originated from the C≡N triple bond in t BuNC. Electron donation from the nitrogen atom to the boron atom in 13-N induced the second Mes migration to the carbon atom to give the aminoboraalkene 14-N . The neutralization of the positively charged Mes group may contribute a large energy gain. A simple coordination of a second t BuNC molecule to 14-N affords the product 5 . This result is consistent with the experimental observation that when t BuNC is in excess the product 5 was obtained. In the absence of excess t BuNC, the boron centre of 14-N would attack to one of the benzylic protons to give the cyclic hydroborate 15-N having delocalized cationic charge on the cyclized Mes ring, as a boryl anion could undergo the same deprotonation cyclization [70] . The energy barrier of 24.2 kcal mol −1 from 14-N to TS15-N is accessible at the room temperature (the reaction condition). Subsequent 1,2-hydride shift from 15-N and re-aromatization would form the product 4 . The formation of B–N π -bond in the last step would contribute a large energy gain. Thus, the detailed spectroscopic and structural analysis of the obtained products and the DFT calculations revealed the complexity of the consecutive rearrangement reactions of 2 . The reason why the newly synthesized diborane(4) 2 showed a remarkable reactivity towards CO and t BuNC in comparison with the conventional boron-containing compounds may be attributed to the existence of two reactive B–C bonds and one reactive B–B bond. Throughout the reactions, the boron atoms in the intermediates undergo repetitive interconversion between sp 2 and sp 3 states to induce the subsequent reactions. In the case of t BuNC, the intermediate 12-N , which is derived after the two π -bonds of the isonitrile moiety have been cleaved, contains a single C–N σ -bond and has a highly nucleophilic nitrogen atom. The highly nucleophilic nitrogen atom facilitates further cleavage of the remaining σ -bond through migrating to the adjacent unsaturated boron centre. Coexistence of the reactive B–B and B–C bonds, steric crowdedness in 2 and the high nucleophilicity of N in 12-N containing a single C–N σ -bond cooperatively achieved the complete cleavage of the C≡N triple bond. In conclusion, we demonstrated the first example of C≡N triple bond cleavage by using newly synthesized diborane(4) 2 in the absence of TM reagents and catalysts. The present results may inspire new idea to achieve multiple bond cleavage reactions using main group element compounds. Accession codes. The X-ray crystal structure information is available at the Cambridge Crystallographic Data Centre (CCDC) under deposition numbers CCDC-985350 ( 1 ), CCDC-981112 ( 2 ), CCDC-981113 ( 3 ), CCDC-981114 ( 4 ), CCDC-981115 ( 5 ) and CCDC-985351 ( 6 ). These data can be obtained free of charge from The Cambridge Crystallographic Data Centre via http://www.ccdc.cam.ac.uk/data_request/cif . How to cite this article: Asakawa, H. et al . Facile scission of isonitrile carbon–nitrogen triple bond using a diborane(4) reagent. Nat. Commun. 5:4245 doi: 10.1038/ncomms5245 (2014).